Mutation within the hinge region of the transcription factorNr2f2attenuates salt-sensitive hypertension Genome-wide association studies (GWAS) have prioritized a transcription factor, nuclear receptor 2 family 2 ( NR2F2 ), as being associated with essential hypertension in humans. Here we provide evidence that validates this association and indicates that Nr2f2 is a genetic determinant of blood pressure (BP). Using the zinc-finger nuclease technology, the generation of a targeted Nr2f2-edited rat model is reported. The resulting gene-edited rats have a 15 bp deletion in exon 2 leading to a five-amino-acid deletion in the hinge region of the mutant Nr2f2 protein. Both systolic and diastolic blood pressures of the Nr2f2 mutant rats are significantly lower than controls. Because the hinge region of Nr2f2 is required for interaction with Friend of Gata2 ( Fog2 ), protein–protein interaction is examined. Interaction of Nr2f2 mutant protein with Fog2 is greater than that with the wild-type Nr2f2, indicating that the extent of interaction between these two transcription factors critically influences BP. Blood pressure (BP) is a complex polygenic trait influenced by multiple genetic elements, the number, magnitude of effect and identities of which are largely unknown. Genome-wide association studies have prioritized genes, on the basis of their association with hypertension, as potential candidates for BP regulation. The Wellcome Trust Case–Control Consortium (WTCCC) was one of the first large scale genome-wide association studies to report a suggestive association on a region on human chromosome 15 to hypertension [1] . Subsequently, by a haplotype-based re-analysis of this data, the gene nuclear receptor subfamily 2, group F, member 2 ( NR2F2 ) also known as chicken ovalbumin upstream promoter transcription factor ( COUP-TFII ) was highly prioritized as a candidate gene associated with hypertension [2] . Four other linkage studies in humans have reported the genomic region containing NR2F2 as being linked to essential hypertension [3] , [4] , [5] , [6] . Similar lines of evidence were obtained with multiple linkage and substitution mapping studies using rat models of hypertension [7] , [8] , [9] , [10] , [11] . Nr2f2 is a nuclear receptor transcription factor vital for angiogenesis and heart development [12] , but its role in BP regulation remains undefined. The current study was conducted to directly test the involvement of Nr2f2 in BP regulation. For this purpose, a targeted gene-edited rat model was generated, in which the Nr2f2 protein was mutated in the hinge region. Both systolic and diastolic BPs of the Nr2f2 mutant rats are significantly lower than controls, indicating that Nr2f2 is indeed a genetic determinant of BP. Further, the structural mechanism by which Nr2f2 influences BP is delineated to the hinge region, through which it interacts with another transcription factor, Friend of Gata2 ( Fog2 ). The extent of interaction of Nr2f2 with Fog2 is enhanced when the Nr2f2 protein is mutated in the hinge region. These data provide evidence for the extent of interaction between two transcription factors, Nr2f2 and Fog2, as being important for the regulation of blood pressure. Targeted-editing of the Nr2f2 locus Gene deletion mouse models serve as genetic tools to validate observations documented through genetic linkage and association studies. Nr2f2 knockout mice are, however, embryonic lethal [13] . To examine the role of Nr2f2 in BP regulation, we therefore focused on constructing a Nr2f2 mutant rat model without disrupting the two important domains of the Nr2f2 protein, the DNA-binding domain and the ligand-binding domain. Custom zinc-finger nucleases (ZFNs) targeting exon 2 of Nr2f2 were designed. Exon 2 of Nr2f2 codes for amino acids in the hinge region of the Nr2f2 protein, which is between the DNA-binding and the ligand-binding domains. ZFNs targeting Nr2f2 were microinjected into single-cell embryos of the hypertensive rat strain—the Dahl salt-sensitive (S) rat. Embryonic lethality was bypassed by the hypomorphic founder Nr2f2 mutant rats. These rats had a shorter (345 bp) PCR-amplified genomic DNA fragment encompassing exon 2 of Nr2f2 compared with the wild-type Nr2f2 (360 bp) genomic fragment ( Fig. 1a ). Sequencing of the PCR products confirmed the deletion to be 15 bp from 1,571 to 1,556 bp of the mRNA of Nr2f2 ( Fig. 1b ). Two different antibodies against Nr2f2 were used to clarify the protein status of Nr2f2. Immunoblotting with an amino (N)-terminal antibody detected the presence of Nr2f2 protein in both the Nr2f2 mutant rats and the wild-type hypertensive rats, whereas antibodies to the hinge region of Nr2f2 cross-reacted exclusively with the wild-type Nr2f2 protein but not the mutant Nr2f2 protein ( Fig. 2 , Supplementary Fig. 1 ). 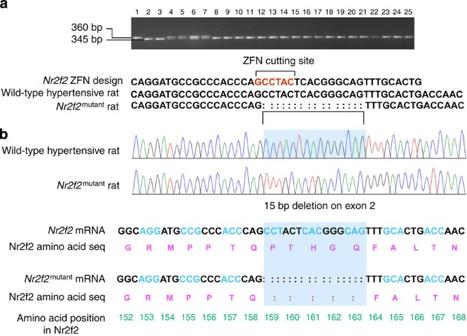Figure 1: Screening animals for ZFN-targeted mutation at theNr2f2locus. (a) Tail DNA samples from pups born post microinjection of custom ZFNs targeting exon 2 of theNr2f2locus were screened by PCR amplification with primers designed to amplify rat genomic fragments encompassing the ZFN-targeted site. Deviations from the expected product size of 360 bp were inferred as genomic DNA from rats with mutations at theNr2f2locus. (b) Representative sequencing results from the PCR products shown inadetected a 15 bp deletion in the mRNA from mutant rats. Also represented are the corresponding translated peptide sequences as a result of the nucleotide variations. Figure 1: Screening animals for ZFN-targeted mutation at the Nr2f2 locus. ( a ) Tail DNA samples from pups born post microinjection of custom ZFNs targeting exon 2 of the Nr2f2 locus were screened by PCR amplification with primers designed to amplify rat genomic fragments encompassing the ZFN-targeted site. Deviations from the expected product size of 360 bp were inferred as genomic DNA from rats with mutations at the Nr2f2 locus. ( b ) Representative sequencing results from the PCR products shown in a detected a 15 bp deletion in the mRNA from mutant rats. Also represented are the corresponding translated peptide sequences as a result of the nucleotide variations. 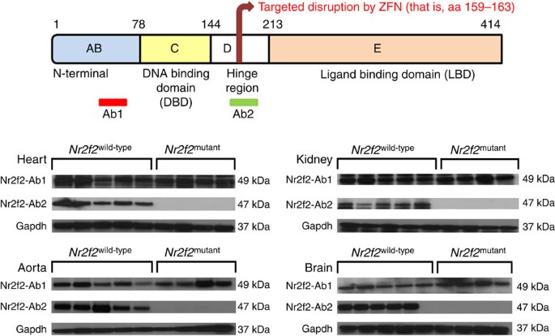Figure 2: Targeted disruption ofNr2f2. Top: Schematic diagram of Nr2f2 protein, highlighting the key domains: AB domain (aa 1–78); C domain or DNA-binding domain (aa 79–144); D domain or hinge region (aa 145–213); E domain or ligand-binding domain (aa 214–414). Bottom: Western blot (WB) analysis of Nr2f2 protein expression inNr2f2mutantand wild-type hypertensive rats. Anti-Nr2f2 antibodies are labelled as Ab1 and Ab2. Ab1: antibody from Abcam, raised against a synthetic peptide directed towards amino acids 43–64 (Abcam); Ab2: antibody (Cell Signaling) raised against a synthetic peptide directed towards the hinge region (amino acids around 159). Full size image Figure 2: Targeted disruption of Nr2f2 . Top: Schematic diagram of Nr2f2 protein, highlighting the key domains: AB domain (aa 1–78); C domain or DNA-binding domain (aa 79–144); D domain or hinge region (aa 145–213); E domain or ligand-binding domain (aa 214–414). Bottom: Western blot (WB) analysis of Nr2f2 protein expression in Nr2f2 mutant and wild-type hypertensive rats. Anti-Nr2f2 antibodies are labelled as Ab1 and Ab2. Ab1: antibody from Abcam, raised against a synthetic peptide directed towards amino acids 43–64 (Abcam); Ab2: antibody (Cell Signaling) raised against a synthetic peptide directed towards the hinge region (amino acids around 159). Full size image Attenuation of hypertension in the Nr2f2 mutant rats Compared with the wild-type hypertensive rats, Nr2f2 mutant rats maintained on a high-salt (2% NaCl) diet had lower systolic BP (179±3 versus 197±5 mm Hg; t -test, P <0.05) as measured by the tail-cuff method. To further confirm these observations, rats were surgically implanted with radio transmitters and BP was continuously recorded by telemetry. Both the Nr2f2 mutant rats and the wild-type hypertensive rats maintained normal diurnal rhythms of systolic and diastolic BP. However, throughout the observation period, both systolic and diastolic BP of the Nr2f2 mutant rats were consistently lower than that of the wild-type hypertensive rats ( Fig. 3a,b ). Nr2f2 mutant rats maintained on a low-salt (0.3% NaCl) diet did not, however, demonstrate a similar BP-lowering effect ( Supplementary Fig. 2 ). 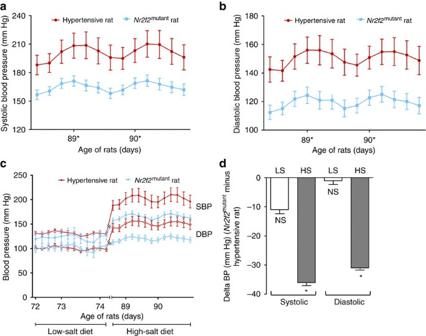Figure 3: Lower blood pressure ofNr2f2mutantrats. Measurements of (a) systolic and (b) diastolic blood pressures of hypertensive rats (n=7) andNr2f2mutantrats (n=8). Rats were monitored for BP after surgical implantation of radiotelemetry transmitters. Data plotted are the recordings obtained once every 5 min continuously for 24 h and averaged for 4 h intervals; (c) Comparison of low-salt versus high-salt diet regimens. Data presented from low-salt and high-salt fed rats were obtained from two independent experiments. (d) Delta BP calculated by subtracting the average BP of the hypertensive rat from the average BP ofNr2f2mutantrats within each of the dietary salt groups labeled as LS for low-salt diet and HS for high-salt diet. Levels of statistical significance for all data were analysed by independent samplet-test. *P<0.05, NS Not significant. Figure 3c,d demonstrate the blunted increase in salt-induced blood pressure in the mutant rats compared with the hypertensive rats. These data constitute strong evidence to indicate that the structural alterations within the hinge region of Nr2f2 contribute importantly to salt-sensitive BP regulation. Figure 3: Lower blood pressure of Nr2f2 mutant rats. Measurements of ( a ) systolic and ( b ) diastolic blood pressures of hypertensive rats ( n =7) and Nr2f2 mutant rats ( n =8). Rats were monitored for BP after surgical implantation of radiotelemetry transmitters. Data plotted are the recordings obtained once every 5 min continuously for 24 h and averaged for 4 h intervals; ( c ) Comparison of low-salt versus high-salt diet regimens. Data presented from low-salt and high-salt fed rats were obtained from two independent experiments. ( d ) Delta BP calculated by subtracting the average BP of the hypertensive rat from the average BP of Nr2f2 mutant rats within each of the dietary salt groups labeled as LS for low-salt diet and HS for high-salt diet. Levels of statistical significance for all data were analysed by independent sample t -test. * P <0.05, NS Not significant. Full size image Improved cardiac and renal function of the Nr2f2 mutant rats Nr2f2 mutant rats exhibited superior cardiac function compared with the wild-type hypertensive rats. As measured by echocardiography, Nr2f2 mutant exhibited superior left ventricular function as demonstrated by increased fractional shortening (FS) (56%±3 versus 41%±2; t -test, P <0.05, Fig. 4a ), increased velocity of circumferential shortening (Vcf) (8.6±0.3 versus 6.1±0.4; t -test, P <0.05, Fig. 4b ) and increased FS/MPI (fractional shortening/myocardial performance index) (1.48±0.22 versus 0.78±0.08; t -test, P <0.05, Fig. 4c ). Nr2f2 mutant rats also exhibited superior renal function compared with the wild-type hypertensive rats. Urinary protein excretion (UPE) of Nr2f2 mutant rats was lower compared with the wild-type hypertensive rats (87.97±7.07 versus 122.63±7.07; t -test, P <0.05; Fig. 5 ). These additional physiological parameters that provide evidence to the overall improvement in cardiovascular and renal function that are associated with the observed lowering of BP in the Nr2f2 mutant rats. 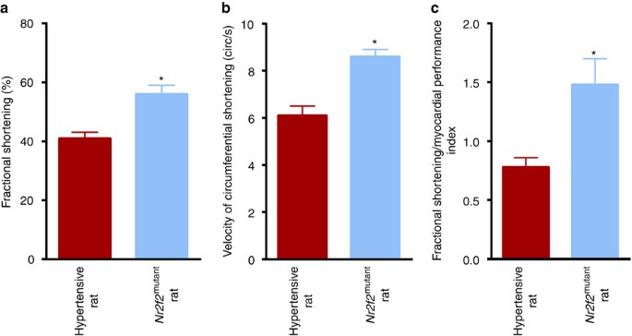Figure 4:Nr2f2mutantrats exhibited superior left ventricular function. Cardiac parameters of male hypertensive rats (n=12) andNr2f2mutantrats (n=12) as determined by echocardiography. (a) Fractional shortening (FS), (b) velocity of circumferential shortening (Vcf) (c) fractional shortening/myocardial performance index (FS/MPI). Levels of statistical significance for all data were analyzed by independent samplet-test; *P<0.05. Figure 4: Nr2f2 mutant rats exhibited superior left ventricular function. Cardiac parameters of male hypertensive rats ( n =12) and Nr2f2 mutant rats ( n =12) as determined by echocardiography. ( a ) Fractional shortening (FS), ( b ) velocity of circumferential shortening (Vcf) ( c ) fractional shortening/myocardial performance index (FS/MPI). Levels of statistical significance for all data were analyzed by independent sample t -test; * P <0.05. 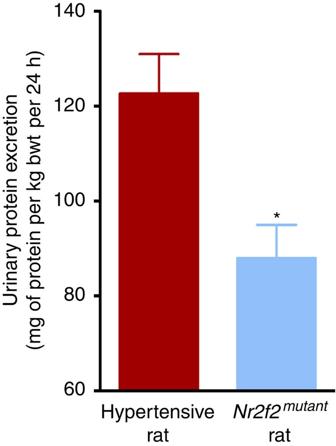Figure 5: Lower urinary protein excretion inNr2f2mutantrats compared with S rats. Total 24 h urine protein was assessed in male hypertensive rats (n=18) andNr2f2mutantrats (n=18) as described in the Methods section. Urinary protein excretion data are presented as milligrams of protein per kg of body weight over a 24 h periodt-test, *P<0.05. Full size image Figure 5: Lower urinary protein excretion in Nr2f2 mutant rats compared with S rats. Total 24 h urine protein was assessed in male hypertensive rats ( n =18) and Nr2f2 mutant rats ( n =18) as described in the Methods section. Urinary protein excretion data are presented as milligrams of protein per kg of body weight over a 24 h period t -test, * P <0.05. Full size image Interaction between Nr2f2 and Fog2 is linked to BP regulation Next, we sought to explore the molecular mechanism by which Nr2f2 mediates the observed alterations in blood pressure and we focused on the sole difference between the two strains, which is in the hinge region of Nr2f2. Amino acids 117–414 of Nr2f2 are required for protein–protein interaction with another transcriptional regulator, Fog2 (ref. 14 ). Fog2 is a multi-zinc-finger transcriptional co-repressor protein required for cardiac development. Fog2 regulates cardiac morphogenesis by interaction with multiple cardiac specific transcriptional factors. Nr2f2 and Fog2 null mice have similar defects related to mesenchymal–epithelial and endothelial interaction, which are important for heart and blood vessel formation [14] . Of further interest, Ciullo et al ., identified a new locus strongly linked to hypertension in human chromosome 8q22–23 region, within which, Fog2 is prioritized as one of the candidate genes for essential hypertension [15] . We therefore hypothesized that the protein–protein interaction between the hinge region of Nr2f2 and Fog2 is important for BP regulation. To test this hypothesis, wild-type and mutant forms of Nr2f2 cDNA, with Histidine tags, were cloned into pCDNA 3.1(B) myc/His (−) expression vector and overexpressed in NRK52E or COS-7 cells ( Fig. 6a , Supplementary Fig. 3 ). The overexpressed Nr2f2 proteins along with their binding partners were immunoprecipitated with the Nr2f2 N-terminal antibody or with histidine tags and probed with the antibody against Fog2. Compared with the wild-type Nr2f2 protein, the binding of the mutant form of Nr2f2 to Fog 2 was more pronounced ( Fig. 6b ). To further assess the downstream effect of this interaction, we conducted a promoter chromatin immunoprecipitation experiment. As shown in Fig. 7 , an enrichment of Nr2f2 binding to the promoter of atrial natriuretic factor, Anf , was noted in the Nr2f2 mutant rats. Anf is a direct target gene known to be influenced by the Nr2f2–Fog2 interaction [14] . Similar enrichments were not observed with promoters for renin and ApoB , which are other targets of Nr2f2 (refs 16 , 17 ) that are not described in the literature to require Fog2. Because Anf is a vasorelaxant [18] , [19] , rats were further tested for vasoreactivity. Vasorelaxation responses of the mesenteric arteries from Nr2f2 mutant rats were significantly higher than that of the wild-type rats ( Fig. 8 ). These data indicate that the extent of interaction between Nr2f2 and Fog2 through the hinge region of Nr2f2 is linked to the extent of blood pressure and that modulation of transcription of Anf , is perhaps, one of the potential underlying mechanisms. 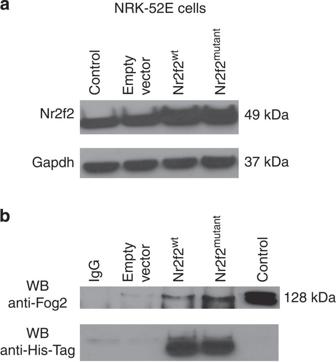Figure 6: Nr2f2 interaction with Fog2. Co-immunoprecipitation analysis of Nr2f2 and Fog2 association in NRK52E cells. Extracts from NRK52E cells were transfected with expression plasmid forNr2f2mutantandNr2f2wildtype. (a) Western blotting (WB) of cell lysates for Nr2f2 protein to confirm the overexpression of both forms of Nr2f2. Lanes labelled from the left—control: NRK52E cell lysate; empty vector: NRK52E cells transfected with empty pcDNA 3.1(-B) myc/His vector; Nr2f2wt: NRK52E cells transfected with Nr2f2 wild-type pcDNA 3.1(B) myc/His (−) construct; Nr2f2mutant: NRK52E cells transfected with Nr2f2 mutant pcDNA 3.1(B) myc/His (−) construct. (b) Cell extracts were subjected to immunoprecipitation (IP) with Nr2f2 antibody (Nr2f2 Ab1). The immune complexes were captured using agarose G beads. The immune-precipitated protein samples were denatured, resolved by SDS–polyacrylamide gel electrophoresis and transferred on to a polyvinylidene difluoride membrane. The membrane was probed by western blotting (WB) with anti-Fog2 antibody and anti-His-Tag antibody. A representative of four experiments is shown. Lanes labelled from the left—IgG: IgG antibody control; empty vector: NRK52E cells transfected with empty pcDNA 3.1(-B) myc/His vector; Nr2f2wt: NRK52E cells transfected with Nr2f2 wild-type pcDNA 3.1(B) myc/His (−) construct; Nr2f2mutant: NRK52E cells transfected with Nr2f2 mutant pcDNA 3.1(B) myc/His (−) construct; control: NRK52E cell lysate. Corroborative data obtained from Histidine-tagged Nr2f2 overexpressed in COS-7 cells are presented inSupplementary Fig. 3. Figure 6: Nr2f2 interaction with Fog2. Co-immunoprecipitation analysis of Nr2f2 and Fog2 association in NRK52E cells. Extracts from NRK52E cells were transfected with expression plasmid for Nr2f2 mutant and Nr2f2 wildtype . ( a ) Western blotting (WB) of cell lysates for Nr2f2 protein to confirm the overexpression of both forms of Nr2f2. Lanes labelled from the left—control: NRK52E cell lysate; empty vector: NRK52E cells transfected with empty pcDNA 3.1(-B) myc/His vector; Nr2f2 wt : NRK52E cells transfected with Nr2f2 wild-type pcDNA 3.1(B) myc/His (−) construct; Nr2f2 mutant : NRK52E cells transfected with Nr2f2 mutant pcDNA 3.1(B) myc/His (−) construct. ( b ) Cell extracts were subjected to immunoprecipitation (IP) with Nr2f2 antibody (Nr2f2 Ab1). The immune complexes were captured using agarose G beads. The immune-precipitated protein samples were denatured, resolved by SDS–polyacrylamide gel electrophoresis and transferred on to a polyvinylidene difluoride membrane. The membrane was probed by western blotting (WB) with anti-Fog2 antibody and anti-His-Tag antibody. A representative of four experiments is shown. Lanes labelled from the left—IgG: IgG antibody control; empty vector: NRK52E cells transfected with empty pcDNA 3.1(-B) myc/His vector; Nr2f2 wt : NRK52E cells transfected with Nr2f2 wild-type pcDNA 3.1(B) myc/His (−) construct; Nr2f2 mutant : NRK52E cells transfected with Nr2f2 mutant pcDNA 3.1(B) myc/His (−) construct; control: NRK52E cell lysate. Corroborative data obtained from Histidine-tagged Nr2f2 overexpressed in COS-7 cells are presented in Supplementary Fig. 3 . 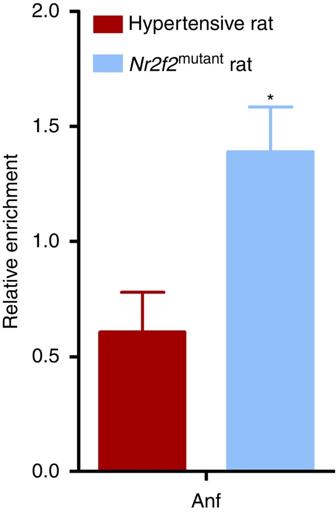Figure 7: Enrichment of Nr2f2 in Anf promoter region inNr2f2mutantrats. Chromatin immunoprecipitation (ChIP) was conducted using heart tissue lysate from wild-type hypertensive (n=3) andNr2f2mutantrats (n=3) with an anti-Nr2f2 antibody (Nr2f2-Ab1, Abcam) or control IgG antibody (Cell signaling). ChIP enrichment at the Anf locus was quantified by qPCR and normalized to haemoglobin (Hbb) promoter amplification, which was used as a negative control. *P<0.05. Full size image Figure 7: Enrichment of Nr2f2 in Anf promoter region in Nr2f2 mutant rats. Chromatin immunoprecipitation (ChIP) was conducted using heart tissue lysate from wild-type hypertensive ( n =3) and Nr2f2 mutant rats ( n =3) with an anti-Nr2f2 antibody (Nr2f2-Ab1, Abcam) or control IgG antibody (Cell signaling). ChIP enrichment at the Anf locus was quantified by qPCR and normalized to haemoglobin ( Hbb ) promoter amplification, which was used as a negative control. * P <0.05. 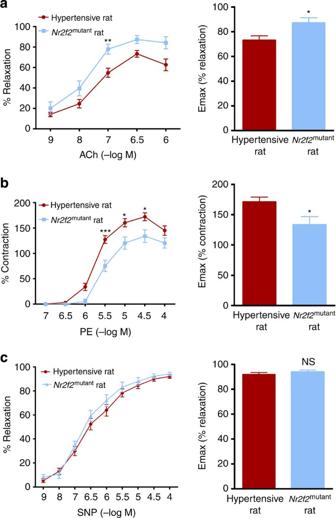Figure 8:Nr2f2mutantrats demonstrated superior vascular function compared with hypertensive rats. (a) Mesenteric arteries from male hypertensive rats (n=9) andNr2f2mutantrats (n=4) were dissected and mounted as described under the Methods section. Endothelium-dependent relaxation to acetylcholine (Ach) was assessed by adding increasing concentrations of ACh (0.001–1 μM) to the vessel preparation. Relaxation to ACh was expressed as a percentage of the level of pre-constriction induced by submaximal dose of phenylephrine. (b) Cumulative concentration-response curves (CCRC) to phenylephrine (0.1–100 μM) of mesentery were recorded from wild-type hypertensive (n=9) andNr2f2mutantrats (n=4). Results are expressed as mean±s.e. (c) Mesenteric arteries from male hypertensive (n=5) andNr2f2mutantrats (n=5) were dissected and mounted as described under the Methods section. Endothelium-independent relaxation to sodium nitroprusside (SNP) was assessed by adding increasing concentrations of SNP (1–100 μM) to the vessel preparation. Relaxation to SNP was expressed as a percentage of the level of pre-constriction induced by submaximal dose of phenylephrine. Data were analysed byt-test. *P<0.05, **P<0.01, ***P<0.001. NS, Not significant. Full size image Figure 8: Nr2f2 mutant rats demonstrated superior vascular function compared with hypertensive rats. ( a ) Mesenteric arteries from male hypertensive rats ( n =9) and Nr2f2 mutant rats ( n =4) were dissected and mounted as described under the Methods section. Endothelium-dependent relaxation to acetylcholine (Ach) was assessed by adding increasing concentrations of ACh (0.001–1 μM) to the vessel preparation. Relaxation to ACh was expressed as a percentage of the level of pre-constriction induced by submaximal dose of phenylephrine. ( b ) Cumulative concentration-response curves (CCRC) to phenylephrine (0.1–100 μM) of mesentery were recorded from wild-type hypertensive ( n =9) and Nr2f2 mutant rats ( n =4). Results are expressed as mean±s.e. ( c ) Mesenteric arteries from male hypertensive ( n =5) and Nr2f2 mutant rats ( n =5) were dissected and mounted as described under the Methods section. Endothelium-independent relaxation to sodium nitroprusside (SNP) was assessed by adding increasing concentrations of SNP (1–100 μM) to the vessel preparation. Relaxation to SNP was expressed as a percentage of the level of pre-constriction induced by submaximal dose of phenylephrine. Data were analysed by t -test. * P <0.05, ** P <0.01, *** P <0.001. NS, Not significant. Full size image In summary, our study provides an important step forward in our current understanding of Nr2f2 as a genetic factor associated with essential hypertension in humans and in rodent models of hypertension. Specifically, combined with the available linkage studies in rat models, by utilizing a novel mutant model of Nr2f2 , we have not only demonstrated that Nr2f2 is a genetic determinant of BP, but also documented the significance of the relatively less-explored hinge region of Nr2f2 as an important molecular feature, which through its interaction with Fog2, is linked to BP regulation. Animals All animal procedures and protocols used in this report were approved by the University of Toledo Health Science Campus Institutional Animal Care and Use Committee. Generation of a ZFN-mediated Nr2f2 mutant rat ZFN construct specific for the rat Nr2f2 gene ( NM_080778.2) were designed, assembled and validated by Sigma-Aldrich, to target the first exon 2 of Nr2f2 (Target sequence: 5′- CAGGATGCCGCCCACCCA gcctac TCACGGGCAGTTTGCACTG -3′; ZFN binds to each underlined sequence on opposite strands). mRNA encoding the Nr2f2 ZFN pairs at a concentration of 10 ng μl −1 were injected into one cell SS/McwiHsd (SS) rat embryos [20] . Out of 147 embryos injected, 66 healthy embryos were transferred to pseudo-pregnant female SD:Crl rats (Charles River), of which five pups were born. At 14 days of age, the pups were tagged, tail clipped and DNA was extracted and amplified using primers flanking the above target sequence Nr2f2 -F (5′-GGGGAAGTGATTTGTGAGGA-3′) and Nr2f2 -R (5′-GCCCATGATGTTGTTAGGCT-3′). PCR products were analysed for ZFN-induced mutations using a Cel-I assay as described previously [20] . Among the five pups born, two positive founders (male/female) were identified. PCR products were TOPO cloned and sequenced to reveal the same 15-bp deletion 5′-CCTACTCACGGGCAG-3′ in exon 2 of the Nr2f2 gene in both mutant animals. The founder male/female rats were backcrossed to the parental SS/JrHsdMcwi strain. Multiple separate pairs of mutation-carrying progeny were then intercrossed to generate an F2 population that was used for phenotyping and breeding to homozygosity. The DNA sequencing of the homozygous Nr2f2 mutant rats confirmed the 15-bp deletion in F2 offspring, which results in a predicted loss of five amino acids PTHGQ. Blood pressure measurements by the tail-cuff and radiotelemetry methods Each set of wild-type hypertensive SS/JrHsdMcwi rats, hitherto referred as hypertensive rats ( n =20 males) and Nr2f2 mutant rats ( n =17 males), hypertensive rats ( n =6 females) and Nr2f2 mutant rats ( n =6 females) were bred, housed and studied concomitantly to minimize environmental effects. All rats were fed with 0.3% NaCl low-salt diet (Harlan Teklad), weaned at 30 days of age. To assess salt sensitivity, at the age of 6 weeks, rats were divided into two groups. The low-salt group was continued to be fed with the 0.3% NaCl low-salt diet, whereas the high-salt group was switched to a diet containing 2% NaCl. After 24 days on these diets, systolic blood pressure (BP) of the rats was measured by using the tail-cuff method [21] . Conscious restrained rats were warmed to 28 °C. The BP of each rat was measured for two consecutive days by two masked operators. BP values for each day were the mean of three or four consistent readings. The final BP value used was the mean of the two daily BP values. BP was also collected using a telemetry system (Data Sciences International, St Paul, MN) [22] . Four days after the BP measurements by the tail-cuff method, Nr2f2 mutant ( n =8 males) and wild-type hypertensive rats ( n =7 males) rats were surgically implanted with C40 radiotelemetry transmitters such that the body of the transmitter is placed into the left flanks and the probe is inserted into their femoral arteries all the way into the lower abdominal aortae. Rats were allowed to recover from surgery for 4 days before the transmitters were turned on for recording BP. Urinary protein excretion Within 5 days following BP measurements, Nr2f2 mutant ( n =17) and wild-type hypertensive ( n =18) rats were housed individually in metabolic cages and urine samples were collected over a 24 h period. The pyrogallol-based QuanTtest Red Total Protein Assay from Quantimetrix (Redondo Beach, CA) was used to determine protein concentrations of the urine samples. A VERSAmax microplate reader from Molecular Devices (Sunnyvale, CA) was used to determine absorbance at 600 nm. Protein concentrations were determined by reading against the absorbance of the QuanTtest human protein standards (25–200 mg dl −1 ). UPE data are presented as milligrams of protein per kg of body weight over a 24 h period (mg of protein per kg bwt per 24 h). Echocardiography Nr2f2 mutant ( n =12) and wild-type hypertensive rats ( n =12) were evaluated by transthoracic echocardiography for the determination of fractional shortening (FS), velocity of circumferential shortening (Vcf), and myocardial performance index(MPI) using a Sequoia C512 System (Siemens Medical) with a 15-MHz linear array transducer [23] , [24] . The rats were anaesthetized with 1.5–2.0% isoflurane by mask, the chest was shaved, the animal was situated in the supine position on a warming pad and ECG limb electrodes were placed. Two-dimensional guided M-mode images and Doppler studies of aortic and trans-mitral flows were obtained from the parasternal long and foreshortened apical windows, respectively. Study duration was typically 15–20 min per animal. All data were analysed offline with software resident on the ultrasound system in an investigator-masked manner. LV end-diastolic (LVDd) and end-systolic (LVSd) dimensions were determined from M-mode tracings recorded at the mid-papillary level, and LV FS was calculated as [(LVDd−LVSd)/LVDd] × 100%. Ejection time and the isovolumic contraction and relaxation times were measured from colour-flow directed Doppler pulsed-wave traces of mitral and aortic flow obtained at the level of the LV outflow tract from the apical four-chamber view. Aortic outflow and mitral inflow waveforms were recorded when the mitral and aortic waveforms were distinct and aortic and mitral valve clicks were clearly visible. Ejection, contraction and relaxation times were determined from three consecutive beats and averaged to calculate MPI. MPI was calculated as the sum of the isovolumic contraction and relaxation times divided by the ejection time. The Vcf was calculated as FS/ejection time. Values are means±s.e.. Groups were compared with Student's t -test. Vascular reactivity After recording blood pressure by radiotelemetry, the wild-type hypertensive ( n =9) and Nr2f2 mutant rats ( n =4) were euthanized with CO 2 inhalation method. The mesentery was immediately excised and placed in ice-cold physiological salt solution (PSS) consisting of mmoles l −1 of 118.5 NaCl, 4.7 KCl, 2.5 CaCl 2 , 1.2 MgSO 4 , 1.2 KH 2 PO 4 , 25.0 NaHCO 3 and 5.5 D -glucose aerated with 95% O 2 –5% CO 2 . Using a dissecting microscope, the mesenteric arteries were gently cleaned of adipose and connective tissue and cut into segments of approximately 2 mm in length. The segments were then mounted in a Mulvany–Halpern style small vessel wire myograph chamber (Model 620M, Danish Myotechnology, Aarhus, Denmark) filled with 6 ml PSS, maintained at 37 °C, and continuously aerated with 95% O 2 , 5% CO 2 to measure vascular reactivity [25] , [26] , [27] . After 30 min of equilibration period, a standardized computer-assisted normalization procedure was performed to set the pretension of the arteries using LabChart8 software (AD Instruments, Colorado Springs, CO). This involves setting a circumference of the arteries equivalent to 90% of that which they would have at a transmural pressure of 100 mm Hg. Segments were washed with PSS and left to equilibrate for another 30 min. Vessel contractility was then assessed with the high-K+ (120 mmol l −1 ) solution. After washing the segment three to four times with PSS, cumulative concentration-response curve to phenylephrine (0.1–100 μM) was obtained. After another 30-min wash, the segments were precontracted with submaximal dose of phenylephrine until the plateau was achieved. Dose-dependent relaxation responses to ACh (0.001–1 μM) and sodium nitroprusside (1 nM–100 μM) were assessed by constructing cumulative concentration-response curve. Relaxation in response to ACh and sodium nitroprusside were expressed as a percentage of the level of pre-constriction induced by submaximal dose of phenylephrine. Western blotting Antibodies were from the following sources: Anti- Nr2f2 mouse monoclonal (Nr2f2-Ab1, Abcam, 1:2,000 dilution), anti-CoupTF II (Nr2f2-Ab2, Cell Signaling, 1:500 dilution), anti-Fog2 (GeneTex, 1:1,000 dilution), donkey anti-mouse IgG-HRP conjugate (SC-2020, 1:5,000 dilution), anti-rabbit IgG-HRP conjugate (Cell Signaling, 1:5,000 dilution). Samples were homogenized in ice-cold RIPA lysis buffer with protease inhibitor cocktail (Pierce). Immunoblotting for Nr2f2 was carried out using tissue lysates from Nr2f2 mutant and wild-type hypertensive rat homogenates. In brief, 40 μg of proteins were boiled with Laemmli sample buffer (Bio-Rad) for 5 min at 95 °C. Protein samples were resolved using 4–15% Criterion Tris-HCl Gel (Bio-Rad) at room temperature, and transferred on to polyvinylidene difluoride membrane (Millipore), blocked with 5% fat-free milk powder in phosphate-buffered saline with Tween 20 and incubated with anti-Nr2f2 and secondary antibodies conjugated with horseradish peroxidase. Immunoreactivity was detected by autoradiography using SuperSignal West Pico Chemiluminescent Substrate (Pierce). Full-length blots are shown in Supplementary Fig. 1 . Chromatin Immunoprecipitation (ChIP) ChIP [16] , [28] was performed using heart tissue from wild-type male hypertensive ( n =3) and Nr2f2 mutant rats ( n =3). Tissues were minced and fixed with 1% formaldehyde. After crosslinking, nuclei were isolated and the cross-linked chromatin was subjected to sonication to obtain DNA fragments. Chromatin (50 μg) was immunoprecipitated with 8 μg of Nr2f2 antibody (Nr2f2-Ab1). As a negative control, chromatin was precipitated with 8 μg of mouse IgG (Cell Signaling). The immune complexes were precipitated with protein G agarose beads. Precipitated chromatin was eluted from the beads and crosslinks were reversed overnight at 65 °C. Chromatin was treated with RNase A, proteinase K and the DNA was column purified (PCR Purification kit, Qiagen). Purified DNA was PCR amplified using primers ( Supplementary Table 1 ) targeting the Anf , Renin and Apob promoter regions, and Hbb used as a negative control. Cell culture, transfection and immunoprecipitation NRK52E cells were obtained from ATCC (Catalogue number CRL-1571) and cultured in DMEM supplemented with 5% fetal bovine serum, 100 units ml −1 penicillin and 100 μg ml −1 streptomycin in a humidified atmosphere at 37 °C with 5% CO 2 . Both wild-type and mutant forms of Nr2f2 cDNA were cloned into the pCDNA 3.1(B) myc/His (−) expression plasmid. NRK52E cells were transfected with both wild-type and mutant forms of Nr2f2 plasmids using X-tremeGENE HP DNA transfection reagent (Roche Applied Science). Forty-eight hours after transient transfection, cells were treated with the cell lysis buffer and used for subsequent experiments. For immunoprecipitation, lysates (500 μg of protein) were pre-cleared with protein G agarose beads (Pierce) at 4 °C for 2 h. After removal of the beads by centrifugation, lysates were incubated overnight with anti-Nr2f2 antibody (5 μg per IP experiment, Nr2f2-Ab1, Abcam) at 4 °C. The immunoprecipitated complex was captured by incubating with 50 μl of protein G agarose beads. Western blotting was performed with Anti-Fog2 antibody (1:1,000 dilution) as detailed above. Statistical analysis All BP statistical analyses were done using the SPSS software (SPSS, Chicago, IL). Data were analysed by independent sample t -test. Data are presented as the mean±standard error. A P value of ≤0.05 was used as a threshold for statistical significance. For BP and UPE experiments measurements, the number of rats in each group ranged from 6 to 20. How to cite this article: Kumarasamy, S. et al . Mutation within the hinge region of the transcription factor Nr2f2 attenuates salt-sensitive hypertension. Nat. Commun. 6:6252 doi: 10.1038/ncomms7252 (2015).